A small molecule restores function to TRPML1 mutant isoforms responsible for mucolipidosis type IV Mucolipidosis type IV (MLIV) is an autosomal recessive lysosomal storage disorder often characterized by severe neurodevelopmental abnormalities and neuro-retinal degeneration. Mutations in the TRPML1 gene are causative for MLIV. We used lead optimization strategies to identify—and MLIV patient fibroblasts to test—small-molecule activators for their potential to restore TRPML1 mutant channel function. Using the whole-lysosome planar patch-clamp technique, we found that activation of MLIV mutant isoforms by the endogenous ligand PI(3,5)P 2 is strongly reduced, while activity can be increased using synthetic ligands. We also found that the F465L mutation renders TRPML1 pH insensitive, while F408Δ impacts synthetic ligand binding. Trafficking defects and accumulation of zinc in lysosomes of MLIV mutant fibroblasts can be rescued by the small molecule treatment. Collectively, our data demonstrate that small molecules can be used to restore channel function and rescue disease associated abnormalities in patient cells expressing specific MLIV point mutations. Mucolipidosis type IV (MLIV) has been described for the first time in the 1970s (ref. 1 ). It is an autosomal recessive lysosomal storage disorder often characterized by severe neurodevelopmental abnormalities, neuro-retinal degeneration and other ophthalmologic signs such as corneal opacity and strabismus. Most patients are unable to speak or walk independently. Storage bodies of lipids and water-soluble substances are seen by electron microscopy in almost every cell type of the patients. Constitutive achlorhydria associated with a secondary elevation of serum gastrin levels is also a characteristic feature of the disease. Iron deficiency anaemia, secondary to the achlorhydria, is another phenotypic feature which occurs in about 50% of the patients [2] , [3] , [4] , [5] . Eventually, mutations in the TRPML1 ( MCOLN1 ) gene were discovered as the genetic cause of MLIV [6] , [7] , [8] . In recent years, TRPML1 has been characterized using electrophysiological tools and its basic cation channel properties have been investigated [9] , [10] , [11] , [12] , [13] , [14] , [15] , [16] , [17] , [18] , [19] , its protein–protein interaction network has been explored [20] , [21] , [22] , [23] , [24] , and knockout mouse models have been generated and investigated [25] , [26] , [27] , [28] . However, effective treatment options for MLIV patients are still missing. Unfortunately, many patients carry mutations that introduce premature stop signals in the TRPML1 gene [6] , [7] , [8] . As a result, the TRPML1 protein is completely absent, or abnormally short and lacks the ion conducting pore between TMD5 and TMD6. Some patients however carry single point mutations which do not destroy the open reading frame [3] , [7] , [29] , [30] , [31] , [32] . While some of these appear to be largely mislocalized, others retain a predominant lysosomal localization. Mutant isoforms that remain or partially remain correctly localized but may be largely inactive on stimulation with endogenous ligands appeared to be good candidates for a small molecule therapeutic approach. An impressive example for such a strategy is the cystic fibrosis transmembrane conductance regulator (CFTR) channel. Here, small-molecule synthetic ligands have recently been developed, which are able to correct the defective gating of, for example, ΔF508-CFTR [33] , [34] . Encouraged by this precedent, we set out for a systematic investigation of small-molecule ligand effects on TRPML1 wild-type- (WT) and mutant-expressing patient fibroblasts. In a translational approach, we studied the potential of these synthetic small-molecule ligands to rescue endogenous channel activity as well as endolysosomal trafficking defects and accumulation of heavy metals (zinc), which may ultimately lead to the observed disease phenotype. Furthermore, by studying the small–molecule-mediated activation of MLIV mutant isoforms such as F465L and F408Δ, we provide novel mechanistic insights into the pH regulation of TRPML1 and synthetic ligand binding. Subcellular localization of MLIV causing TRPML1 mutants To analyse the subcellular localization of TRPML1 mutant channels, YFP-tagged hTRPML1 WT and mutant channels were expressed in murine embryonic fibroblasts and colocalization of channel proteins with lysosomes was visualized using LysoTracker Deep Red. We focused on several MLIV causing point mutants described in the literature with either unknown subcellular localization (R403C, Y436C, V446L, V447P, S456L) [3] , [7] , [29] , [31] , [32] , or mutant isoforms reported to show partial localization on endosomes and lysosomes, that is, F408Δ, an in-frame mutant that lacks one amino acid, and F465L [7] , [30] ( Fig. 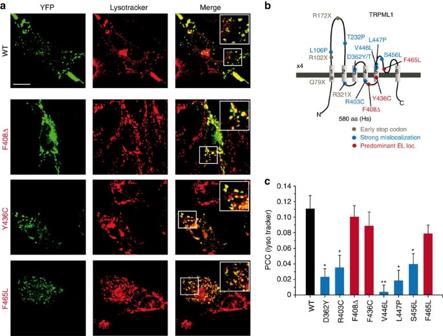Figure 1: Subcellular localization of MLIV causing point mutants of TRPML1. (a) Representative images of WT and selected MLIV causing mutant isoforms of human TRPML1 overexpressed in WT fibroblasts. Depicted mutants show predominant endolysosomal localization. All WT and mutant variants were cloned with YFP in fusion at the C terminus. Cells were transfected for 24–48 h and incubated with LysoTracker Deep Red (100 nM) for 30 min at 37 °C before confocal analysis. Scale bar, 20 μm. (b) Cartoon of the human TRPML1 protein illustrating the estimated positions of known MLIV causing TRPML1 point mutations in exon regions. (c) Pearson Correlation Coefficients (PCC) to quantify the colocalization of TRPML1 WT and mutant isoforms with LysoTracker Deep Red. Shown are mean PCC values±s.e.m. of at least 10 cells, each; **P<0.01, *P<0.05. Statistical significance was determined via one-way analysis of variance followed by Tukey’s post test. 1a,b ; Supplementary Table 1 ; Supplementary Fig. 1 ). We confirmed substantial colocalization of LysoTracker with TRPML1-YFP WT. We further found that F408Δ, Y436C and F465L show substantial colocalization with LysoTracker ( Fig. 1a ). R403C, V446L, V447P and S456L did colocalize to a much lesser extent with LysoTracker compared with WT and rather showed an expression pattern similar to L106P or D362Y, reported previously to colocalize with the ER [35] , [36] . To quantify the relative degree of colocalization between LysoTracker and TRPML1 or the MLIV mutants, we calculated the respective Pearson Correlation Coefficients ( Fig. 1c ). Figure 1: Subcellular localization of MLIV causing point mutants of TRPML1. ( a ) Representative images of WT and selected MLIV causing mutant isoforms of human TRPML1 overexpressed in WT fibroblasts. Depicted mutants show predominant endolysosomal localization. All WT and mutant variants were cloned with YFP in fusion at the C terminus. Cells were transfected for 24–48 h and incubated with LysoTracker Deep Red (100 nM) for 30 min at 37 °C before confocal analysis. Scale bar, 20 μm. ( b ) Cartoon of the human TRPML1 protein illustrating the estimated positions of known MLIV causing TRPML1 point mutations in exon regions. ( c ) Pearson Correlation Coefficients (PCC) to quantify the colocalization of TRPML1 WT and mutant isoforms with LysoTracker Deep Red. Shown are mean PCC values±s.e.m. of at least 10 cells, each; ** P <0.01, * P <0.05. Statistical significance was determined via one-way analysis of variance followed by Tukey’s post test. Full size image SF-22 increases channel activity of TRPML1 mutant isoforms We have previously reported that a plasma membrane variant (PM variant) of WT hTRPML1 (TRPML1ΔNC) can be activated by SF-22 (5-chloro- N -(2-piperidin-1-ylphenyl)thiophene-2-sulphonamide) in calcium imaging experiments [15] . Here, we applied the whole-lysosome planar patch-clamp technique [37] , [38] to investigate the small-molecule activation of WT hTRPML1 and selected mutant isoforms of TRPML1. We demonstrate that SF-22 elicits inwardly rectifying (from lysosomal lumen to cytosol) currents in lysosomes isolated from a HEK293 cell line stably expressing hTRPML1 ( Fig. 2a ). We further show that PI(3,5)P 2 , which has been reported recently to activate TRPML channels [14] , has a comparable effect on TRPML1 channel activity as SF-22 when applied at a concentration of 10 μM, respectively ( Fig. 2b ). Both, SF-22 and PI(3,5)P 2 evoked currents were reduced when luminal pH was increased as reported previously ( Fig. 2a,b ; SF-22: −43.1±3.9 pA ( n =3; pH 7.2) versus −107.4±10.6 pA ( n =9; pH 4.6) at −200 mV; PI(3,5)P 2 : −28±2 pA ( n =4; pH 7.2) versus −101.7±9.2 pA ( n =7; pH 4.6) at −200 mV) (refs 9 , 16 ). We further show that the observed effects are independent of the compound applied to increase the size of the lysosomes before isolation and patch-clamp experimentation. Both, treatment with vacuolin or the PIKfyve inhibitor YM-201636 showed similar results ( Supplementary Fig. 2 ). 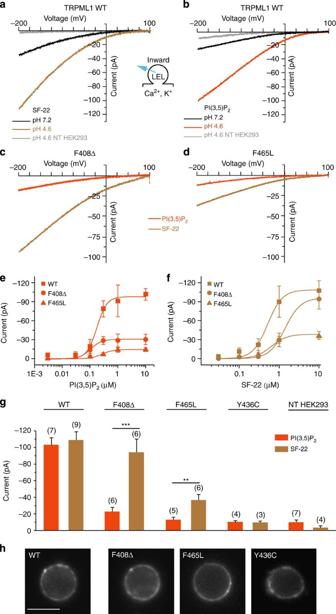Figure 2: Effect of small-molecule activators and PI(3,5)P2on activation of TRPML1 WT and mutant channel isoforms overexpressed in HEK293 cells. (a,b) Current–voltage relations of whole-lysosome planar patch-clamp experiments demonstrating that human TRPML1-YFP is activated by SF-22 (10 μM) (a) and PI(3,5)P2(diC8, 10 μM) (b) in a pH-dependent manner; NT, non-transfected control cells (c,d) Current–voltage relations of whole-lysosome planar patch-clamp experiments demonstrating that the effect of PI(3,5)P2on the channel activity of MLIV causing TRPML1 mutant isoforms F408Δor F465L is three to fourfold smaller than the effect of SF-22. (e,f) Dose–response curves showing effects of SF-22 and PI(3,5)P2on mutant and WT TRPML1 expressing lysosomes. (g) Bar diagram summarizing data at −200 mV from experiments shown ina–d. ***P<0.001, **P<0.01;n=number of experiments. (h) Fluorescence images of enlarged lysosomes isolated from TRPML1 mutant and WT-expressing HEK293 cells after vacuolin treatment. Scale bar, 5 μm. Figure 2: Effect of small-molecule activators and PI(3,5)P 2 on activation of TRPML1 WT and mutant channel isoforms overexpressed in HEK293 cells. ( a , b ) Current–voltage relations of whole-lysosome planar patch-clamp experiments demonstrating that human TRPML1-YFP is activated by SF-22 (10 μM) ( a ) and PI(3,5)P 2 (diC8, 10 μM) ( b ) in a pH-dependent manner; NT, non-transfected control cells ( c , d ) Current–voltage relations of whole-lysosome planar patch-clamp experiments demonstrating that the effect of PI(3,5)P 2 on the channel activity of MLIV causing TRPML1 mutant isoforms F408Δor F465L is three to fourfold smaller than the effect of SF-22. ( e , f ) Dose–response curves showing effects of SF-22 and PI(3,5)P 2 on mutant and WT TRPML1 expressing lysosomes. ( g ) Bar diagram summarizing data at −200 mV from experiments shown in a – d . *** P <0.001, ** P <0.01; n =number of experiments. ( h ) Fluorescence images of enlarged lysosomes isolated from TRPML1 mutant and WT-expressing HEK293 cells after vacuolin treatment. Scale bar, 5 μm. Full size image When PI(3,5)P 2 was applied on lysosomes overexpressing the mutant isoforms F408Δ, Y436C or F465L, we found that its effect on channel activity was much smaller compared with WT. Surprisingly, SF-22 evoked channel activity in F408Δ and F465L lysosomes was three to fourfold higher compared with PI(3,5)P 2 ( Fig. 2c,d,h ). Dose–response measurements with PI(3,5)P 2 revealed a strong decrease in efficacy for both F408Δ and F465L compared with WT, while EC 50 values (relative potency) were comparable (0.17±0.01 μM for WT TRPML1, 0.27±0.14 μM for F465L and 0.1±0.03 μM for F408Δ) ( Fig. 2e ). Dose–response measurements with SF-22 revealed an EC 50 of 0.51±0.05 μM for WT TRPML1, 0.64±0.17 μM for F465L and 1.41±0.36 μM for F408Δ. While F408Δ showed a significant shift in the dose–response curve affecting potency, the relative efficacy of SF-22 was similar in F408Δ compared with WT. In contrast, it was decreased in F465L ( Fig. 2f,g ). No significant channel activation could be detected with SF-22 on lysosomes expressing the Y436C mutant although Y436C was present in LysoTracker positive vesicles in intact cells as well as in enlarged isolated lysosomes ( Figs 1b and 2h ). Further development of the lead structure SF-22 With the aim to further improve the efficacy and potency profile of SF-22, we generated several series of chemically modified SF-22 analogues ( Fig. 3a and Supplementary Figs 3 and 4 ) and analysed them using single-cell calcium imaging and the PM variant of TRPML1 (TRPML1(NC)) [15] ( Fig. 3b ; Supplementary Fig. 3 ). Systematic modifications were performed in any structural motif of the lead structure (phenyl ring, thiophene, piperidine and sulphonamide; n =40 compounds/modifications total) ( Fig. 3a ). 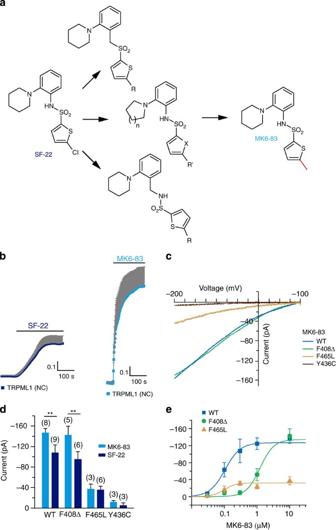Figure 3: Screening for novel SF-22 analogues and effect of SF-22 and MK6-83 on TRPML1 channel activity in WT- and mutant isoform-expressing lysosomes. (a) Shown are the main strategies of chemical modifications of SF-22 and the chemical structure of the novel lead compound MK6-83. For further details, refer toSupplementary Methodssection andSupplementary Figs 3 and 4. (b) Shown are representative calcium imaging measurements of HEK293 cells transiently transfected with the PM variant TRPML1(NC)-YFP and loaded with fura-2 (mean values±s.e.m. of at least 10 cells, each). (c) Current–voltage relations of whole-lysosome planar patch-clamp experiments demonstrating activation of hTRPML1 and MLIV causing mutant isoforms by MK6-83 (10 μM). (d) Bar diagram summarizing data at −200 mV from experiments shown in a in comparison to SF-22 effects. (e) Dose–response curves showing potency of MK6-83 on TRPML1 WT- and mutant isoform-expressing lysosomes. Figure 3: Screening for novel SF-22 analogues and effect of SF-22 and MK6-83 on TRPML1 channel activity in WT- and mutant isoform-expressing lysosomes. ( a ) Shown are the main strategies of chemical modifications of SF-22 and the chemical structure of the novel lead compound MK6-83. For further details, refer to Supplementary Methods section and Supplementary Figs 3 and 4 . ( b ) Shown are representative calcium imaging measurements of HEK293 cells transiently transfected with the PM variant TRPML1(NC)-YFP and loaded with fura-2 (mean values±s.e.m. of at least 10 cells, each). ( c ) Current–voltage relations of whole-lysosome planar patch-clamp experiments demonstrating activation of hTRPML1 and MLIV causing mutant isoforms by MK6-83 (10 μM). ( d ) Bar diagram summarizing data at −200 mV from experiments shown in a in comparison to SF-22 effects. ( e ) Dose–response curves showing potency of MK6-83 on TRPML1 WT- and mutant isoform-expressing lysosomes. Full size image In calcium imaging experiments, we found that modifying the thiophene rest in SF-22 by replacing chlorine with a methyl group (MK6-83) greatly increased compound efficacy for TRPML1 while other modifications were not beneficial ( Fig. 3b ; Supplementary Fig. 3 ). In lysosomal planar patch-clamp experiments we confirmed that, compared with SF-22, MK6-83 showed an increased efficacy in activating TRPML1 WT and F408Δ in isolated lysosomes. Efficacy remained unaltered in F465L lysosomes ( Fig. 3c–e ). Likewise, unaltered efficacy was seen in Y436C-expressing lysosomes ( Fig. 3c–e ). Next, we performed dose–response measurements that revealed an EC 50 of 0.11±0.01 μM for WT TRPML1 and 0.1±0.03 μM for F465L when activated with MK6-83 ( Fig. 3e ) compared with 0.51±0.05 μM for WT TRPML1 and 0.64±0.17 μM for F465L when activated with SF-22 ( Fig. 2f ). Thus, compound MK6-83 showed improved potency in WT and F465L lysosomes, while potency was not significantly shifted in F408Δ lysosomes (1.23±0.19 μM versus 1.41±0.36 μM for SF-22) ( Fig. 3e ). We further found that F465L is insensitive to pH changes when activated with SF-22 or MK6-83 (pH 4.6 luminal versus pH 7.2 luminal), while F408Δ shows similar pH sensitivity as WT TRPML1 ( Fig. 4a–c ). The effects of synthetic and endogenous ligands (SF-22 and PI(3,5)P 2 ) were additive, suggesting different binding sites and independent gating mechanisms, while the effects of the two structurally related sythetic ligands SF-22 and MK6-83 were not additive, most likely due to competition for the same binding site ( Fig. 4d–h ). 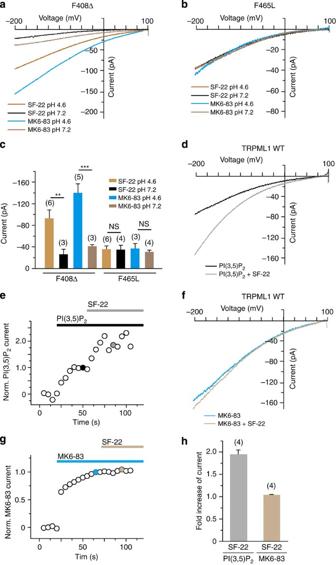Figure 4: Regulation of TRPML1 mutant isoforms by pH and additive effect between endogenous and synthetic TRPML1 ligands. (a) Similar to the WT channel activity of TRPML1 mutant isoform F408Δ is enhanced by low pH. (b) Lack of effect of low pH on F465L. (c) Bar diagram summarizing data at −200 mV from experiments shown ina,b. (d,e) Additive effect of PI(3,5)P2and SF-22 on WT TRPML1 currents in lysosomes (d) and respective time course of current shown ind(e). (f,g) Lack of additive effect after co-application of SF-22 and MK6-83 (f) and respective time course of current shown inf(g). (h) Bar diagram summarizing data from experiments shown ind,g. ***P<0.001, **P<0.01;n=number of experiments. Data are presented as mean±s.e.m. Figure 4: Regulation of TRPML1 mutant isoforms by pH and additive effect between endogenous and synthetic TRPML1 ligands. ( a ) Similar to the WT channel activity of TRPML1 mutant isoform F408Δ is enhanced by low pH. ( b ) Lack of effect of low pH on F465L. ( c ) Bar diagram summarizing data at −200 mV from experiments shown in a , b . ( d , e ) Additive effect of PI(3,5)P 2 and SF-22 on WT TRPML1 currents in lysosomes ( d ) and respective time course of current shown in d ( e ). ( f , g ) Lack of additive effect after co-application of SF-22 and MK6-83 ( f ) and respective time course of current shown in f ( g ). ( h ) Bar diagram summarizing data from experiments shown in d , g . *** P <0.001, ** P <0.01; n =number of experiments. Data are presented as mean±s.e.m. Full size image To test for cell viability, we performed MTT (3-[4,5-dimethylthiazol-2-yl]-2,5-diphenyl-tetrazolium bromide) tests [39] . We used plumbagin (5-hydroxy-2-methyl-1,4-naphthoquinone) and the protein kinase inhibitor staurosporine as positive controls to demonstrate cell toxicity and found that concentrations of MK6-83 and SF-22 ranging from 0.2 to 30 μM showed no signs of cytotoxicity ( Supplementary Fig. 5 ). In summary, the above-described chemical modifications led to a new candidate activator of TRPML1 with an improved efficacy and potency profile: MK6-83. Effect of SF-22 and MK6-83 on MLIV patient-derived cells To test for in vivo effects of the TRPML1-activating compounds, we persued a translational approach. We used lysosomes isolated from fibroblast cell lines derived from MLIV patients carrying either the F408Δ, the R403C or the V446L mutation. Human TRPML1 +/+ (GM03440) and TRPML1 −/− (GM02048) fibroblast cell lines were used as positive and negative control, respectively. In line with the above-described results for overexpressing HEK293 cells, we found that lysosomes isolated from TRPML1 +/+ fibroblasts (WT) were activated by SF-22 and MK6-83. As further expected, MK6-83 showed greater efficacy than SF-22 ( Fig. 5a,f,g ). Lysosomes isolated from F408Δ expressing cells showed activation similar to WT for both compounds ( Fig. 5b,f,g ). In contrast, SF-22 and MK6-83 had no significant effect on lysosomes isolated from TRPML1 −/− fibroblasts ( Fig. 5c,f,g ). Lysosomes isolated from R403C or V446L expressing cells showed only little activation by SF-22 and MK6-83. Nevertheless, MK6-83 appeared to be significantly more efficacious on fibroblast lysosomes isolated from R403C or V446L expressing cells than on those isolated from TRPML1 −/− cells ( Fig. 5d,e,g ). 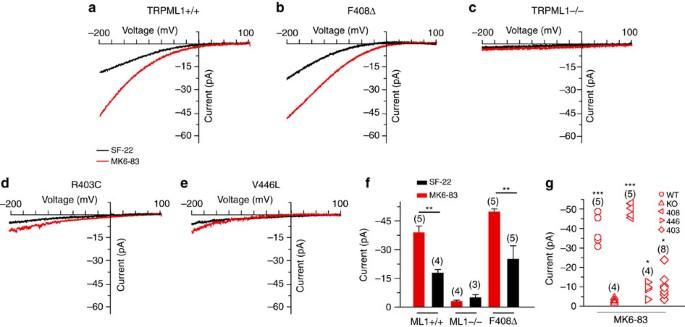Figure 5: SF-22 and MK6-83 evoked currents in human patient fibroblasts. (a–e) Representative currents elicited in lysosomes isolated from human fibroblast cells derived from healthy individuals (a) Individuals with MLIV causing mutations in TRPML1 resulting in the complete loss of TRPML1 protein (TRPML1−/−) (b) or individuals with MLIV causing point mutations in TRPML1: V446L (c) F408Δ (d) and R403C (e). (f) Bar diagram summarizing data at −200 mV from experiments shown ina–c. Recordings shown were obtained with 10 μM SF-22 and 10 μM MK6-83, respectively. (g) Dot plot summarizing data at −200 mV from experiments shown ina–e. Recordings shown were obtained with 10 μM MK6-83, respectively. ***P<0.001, **P<0.01, *P<0.05;n=number of experiments. Data are presented as mean±s.e.m. Figure 5: SF-22 and MK6-83 evoked currents in human patient fibroblasts. ( a – e ) Representative currents elicited in lysosomes isolated from human fibroblast cells derived from healthy individuals ( a ) Individuals with MLIV causing mutations in TRPML1 resulting in the complete loss of TRPML1 protein (TRPML1 −/− ) ( b ) or individuals with MLIV causing point mutations in TRPML1: V446L ( c ) F408Δ ( d ) and R403C ( e ). ( f ) Bar diagram summarizing data at −200 mV from experiments shown in a – c . Recordings shown were obtained with 10 μM SF-22 and 10 μM MK6-83, respectively. ( g ) Dot plot summarizing data at −200 mV from experiments shown in a – e . Recordings shown were obtained with 10 μM MK6-83, respectively. *** P <0.001, ** P <0.01, * P <0.05; n =number of experiments. Data are presented as mean±s.e.m. Full size image MK6-83 effects on trafficking and lysosomal zinc buildup Lactosylceramide has been used before to demonstrate abberrant trafficking in MLIV fibroblasts [40] , [41] , [42] , [43] . In the present study, we used BODIPY FL C5-LacCer and examined its distribution in WT and MLIV fibroblasts in pulse-chase experiments. In MLIV cells, a strong punctate pattern of LacCer was observed across the cell soma, while in WT cells a predominant perinuclear pattern of LacCer was found with little labelling of cytoplasmic vesicles as described previously [40] , [41] ( Fig. 6a ). Like TRPML1 −/− , F408Δ mutant-expressing fibroblasts presented with prominent labelling of cytoplasmic vesicles ( Fig. 6a ). Treatment with MK6-83 but not with solvent only (dimethyl sulfoxide (DMSO)) for 24 h led to an efficient rescue of the trafficking defects in F408Δ mutant channel-expressing cells. In contrast, no effect was found on TRPML1 −/− cells ( Fig. 6a,b ). 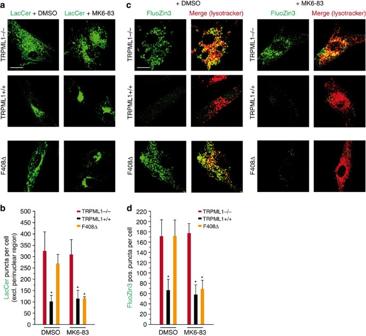Figure 6: Rescue effect of MK6-83. (a,b) Effects of 10 μM DMSO or MK6-83 on BODIPY FL C5-LacCer trafficking in human patient fibroblasts. Shown are the representative cells ina. Quantification is shown inb: mean values±s.e.m. of at least 20 cells from three independent experiments; *P<0.05. Statistical significance was determined via one-way analysis of variance followed by Tukey’s post test. (c) Effects of 10 μM DMSO or MK6-83 on lysosomal zinc accumulation in human patient fibroblasts. (d) Quantification of experiments as shown in c. Figure 6: Rescue effect of MK6-83. ( a , b ) Effects of 10 μM DMSO or MK6-83 on BODIPY FL C5-LacCer trafficking in human patient fibroblasts. Shown are the representative cells in a . Quantification is shown in b : mean values±s.e.m. of at least 20 cells from three independent experiments; * P <0.05. Statistical significance was determined via one-way analysis of variance followed by Tukey’s post test. ( c ) Effects of 10 μM DMSO or MK6-83 on lysosomal zinc accumulation in human patient fibroblasts. ( d ) Quantification of experiments as shown in c. Full size image Different groups have previously reported that zinc accumulates in lysosomes in MLIV fibroblasts or after knockdown of TRPML1 [44] , [45] . Heavy metal accumulation may ultimately lead to the neurodegenerative effects seen in MLIV patients. We used MLIV fibroblasts to verify these findings and to examine a possible rescue effect of MK6-83 on lysosomal zinc accumulation. We found that LysoTracker positive compartments of TRPML1 −/− fibroblasts displayed strong vesicular FluoZin-3 fluorescence when pretreated with ZnCl 2 as described previously [45] , [46] . The zinc accumulation in TRPML1 −/− fibroblasts was not reversible on treatment with MK6-83. In contrast, zinc accumulation in F408Δ mutant-expressing cells was significantly ameliorated by MK6-83 ( Fig. 6c,d ). Not only the number but also the size of FluoZin-3 positive structures was markedly reduced and comparable to WT. In the present study, we developed a novel small-molecule agonist of TRPML1, termed MK6-83. Using this agonist, we demonstrate that the effect of specific MLIV causing mutations on TRPML1 channel activity and its functions in endolysosomal trafficking and heavy metal homeostasis can be restored. While the synthetic ligand strongly activates WT and the mutant isoforms F408Δ and F465L, channel activation by its endogenous ligand PI(3,5)P 2 is remarkably reduced in these mutants. F408 resides at the lower end of TMD4 or shortly after TMD4, depending on the applied prediction programme. F465 is part of the highly conserved pore helix region. The obtained potency data suggest that loss of phenylalanine at position F408 has an effect on the binding affinity of small molecule ligands of the SF-22 type, while the change in efficacy in case of F465L points to a change in the ability of the compound to produce the same maximal response as in the WT isoform, possibly due to severe alterations in the pore region of the channel. Notably, we found that F465L has lost its pH sensitivity. Loss of phenylalanine at position 465 abrogates the proton-mediated increase in channel activity observed in WT TRPML1. We thus provide novel mechanisitic insights into the pH regulation of TRPML1. Critical sites for pH regulation have been found in other TRP channels to reside in the pore region, for example, in case of TRPV1 (refs 47 , 48 ). For example, amino acid F660 has recently been identified as essential for the proton-mediated gating of TRPV1 (ref. 48 ). Interestingly, none of the test compounds could evoke significant channel activation in Y436C-expressing lysosomes although Y436C, just like F408Δ and F465L, appears to still largely reside in lysosomes ( Fig. 1a ). Y436C is located in the centre of TMD5 of TRPML1. TMD5 mutations in TRPML channels have recently been shown to have a critical impact on TRPML channel opening (varitint-waddler mutant isoforms and analogues). Thus, mutation of V432 to proline renders TRPML1 constitutively active [10] , [13] . Likewise, C430P and C431P mutants were found to be constitutively active. In contrast, V436P rendered the channel completely inactive [13] . Similarly, V436C may render the channel inactive by a mechanism which cannot be overcome by compounds of the SF-22 type. Most importantly, in a translational approach, we found that the small-molecule agonists of TRPML1 have the ability to restore channel activity in lysosomes isolated from MLIV patient fibroblasts and to improve defects in endolysosomal trafficking (LacCer) as well as heavy metal ion homeostasis (lysosomal zinc accumulation) observed in MLIV mutant cells. While MK6-83 had a significant rescue effect on F408Δ mutant-expressing fibroblasts, LacCer trafficking could not be rescued in cells completely lacking expression of TRPML1 (TRPML1 −/− ). Similar to the LacCer trafficking defect, we found that zinc accumulation in TRPML1 −/− fibroblasts was not reversible on treatment with MK6-83. In contrast, zinc accumulation in F408Δ mutant-expressing cells was strongly reduced by MK6-83. In summary, the results suggest that the novel TRPML1 activator MK6-83 may be used as a potential pharmacological treatment option for a specific subgroup of MLIV patients. Compounds and chemical syntheses Compounds SF-22 (ref. 15 ) and Z133963852 (5-chloro- N -methyl- N -{[2-(piperidin-1-yl)phenyl]methyl} thiophene-2-sulphonamide) were purchased through MolPort (MolPort, Latvia): MolPort-004-039-979 (SF-22) and MolPort-009-399-330 (Z133963852). Stock solutions of 10 mM in DMSO were prepared for each compound. All other compounds were synthesized de novo as described in the Supplementary Methods section. Briefly, the sulphonamides were obtained from the amine building blocks (ring-substituted anilines, aminopyridines, cyclohexylamines, benzylamines) and appropriate thiophene (or furan) sulfonyl chlorides. The thiophenecarboxamides were obtained in an analogous manner from the appropriate carboxylic acid chlorides. The thienyl sulphones were obtained by alkylation of sodium sulfinates (prepared by reduction of sulfonyl chlorides) with an appropriate benzyl chloride. cDNA constructs, cell culture and transfection Human WT TRPML1 was subcloned into pcDNA3 expression vector (Invitrogen Life Technologies, Breda, The Netherlands) as described before [15] . All point mutations were generated by standard QuikChange site-directed mutagenesis according to the manufacturer’s guidelines (Agilent Technologies Inc., USA). HEK293 cells were maintained in Dulbecco’s Modified Eagle Medium (DMEM) supplemented with 10% fetal bovine serum (FBS), 100 U penicillin per ml and 100 μg streptomycin per ml. HEK293 cells were transiently transfected with Fugene (Roche) or GeneExpresso Max Transfection Reagent (Excellgen) according to the manufacturer’s protocols and used for LSM experiments 24–48 h after transfection. Murine embryonic fibroblasts were maintained in DMEM supplemented with 10% FBS, 100 U penicillin per ml and 100 μg streptomycin per ml. Cells were transiently transfected with TurboFect (Fermentas) according to the manufacturer’s protocol and used for further processing 24–48 h after transfection. Human skin fibroblast cells from a MLIV patient (TRPML1 −/− , clone GM02048) and a WT control (TRPML1 +/+ , clone GM03440) were obtained from the Coriell Institute for Medical Research (NJ, USA). Other human fibroblast cell lines were provided by Dr Schiffmann (Institute of Metabolic Disease, Baylor Research Institute, Dallas, TX, USA). All human material was obtained and worked with in compliance with ethical regulations. Planar patch-clamp electrophysiology and calcium imaging Whole-lysosome planar patch-clamp recordings and preparation of lysosomes (HEK293, Human Fibroblast) were performed as described previously [37] , [38] . In brief, late endosomes and lysosomes were enlarged by treating the cells with 1 μM vacuolin-1 overnight [12] , [37] , [38] , [49] . The following day, cells were homogenized in homogenization buffer (0.25 M sucrose, 10 mM Tris-Cl, pH 7.4) on ice using a potter homogenizer to obtain whole-cell lysates. The lysates were centrifuged at 14,000 g for 15 min at 4 °C. The supernatant was treated with 8 mM CaCl 2 (final concentration) on ice for 5 min, followed by a second centrifugation step at 25,000 g for 15 min at 4 °C. The supernatant was collected and the pellet washed in 150 mM KCl, 10 mM Tris-Cl, pH 7.4, followed by a final centrifugation step at 25,000 g for 15 min at 4 °C. The planar patch-clamp technology combined with a pressure control system and microstructured glass chips containing an aperture of ~1 μm diameter (resistances of 10–15 MΩ) (Port-a-Patch, Nanion Technologies) were applied as described [37] , [38] . Currents were recorded using an EPC-10 patch-clamp amplifier and PatchMaster acquisition software (HEKA). Data were digitized at 40 kHz and filtered at 2.8 kHz. Cytoplasmic solution contained (in mM) 60 KF, 70 K-MSA (methanesulfonate), 0.2 Ca-MSA, 10 HEPES (pH adjusted with KOH to 7.2). Luminal solution was 60 Ca-MSA, 70 K-MSA, 10 HEPES (pH adjusted with MSA to 4.6). The membrane potential was held at +60 mV, and 500 ms voltage ramps from −200 to +100 mV were applied every 5 s. Due to high luminal calcium used to ensure giga seals when performing whole-endolysosomal patch-clamp on the port-a-patch system [37] , [38] , the inward currents are less rectifying and reverse at more positive potentials, depending on current amplitude and protein expression level [9] . All recordings were obtained at room temperature and were analysed using PatchMaster (HEKA) and Origin 6.1 (OriginLab) software. Liquid junction potential was corrected. Water-soluble diC8-PIP 2 , PI(3,5)P 2 were purchased from A.G. Scientific. No significant differences in TRPML1 channel properties were seen for recordings obtained with full-length diC16 PI(3,5)P 2 and diC8 PI(3,5)P 2 (ref. 14 ). For the application of all activators, cytoplasmic (external) solution was completely exchanged by a solution containing the respective activator. The EC 50 values of graded dose–response curves were fitted with the Hill equation. Calcium imaging experiments were performed using fura-2 as described previously. Briefly, HEK293 cells were plated onto glass coverslips, grown over night and transiently transfected with the respected cDNAs using TurboFect transfection reagent (Thermo Scientific). After 24–48 h, cells were loaded for 1 h with the fluorescent indicator fura-2-AM (4 μM; Invitrogen) in a standard bath solution containing (in mM) 138 NaCl, 6 KCl, 2 MgCl 2 , 2 CaCl 2 , 10 HEPES and 5.5 D -glucose (adjusted to pH 7.4 with NaOH). Cells were washed in standard bath solution for 30 min before measurement. Calcium imaging was performed using a monochromator-based imaging system (Polychrome IV monochromator, TILL Photonics). Lactosylceramide trafficking assay Human WT, knockout and mutant TRPML1 fibroblasts were grown in Poly- D -Lysine-coated 1 μ–Slide 8 wells (ibidi, Germany) and were treated for 24 h with DMSO or MK6-83 (in DMSO) at a final concentration of 10 μM, respectively. Cells were washed with PBS and then incubated with 5 μM LacCer (BODIPY FL C5-Lactosylceramide (Invitrogen), prepared according to manufacturer’s instructions) in serum-free DMEM for 1 h at 37 °C, in the presence of DMSO or MK6-83. Cells were washed twice with PBS and then incubated with normal DMEM (with 10% FBS) for 1 h at 37 °C. Cells were washed again with PBS and immediately analysed using a Zeiss Confocal microscope (LSM 510). For data quantification ImageJ software was used. In each experiment, numbers were calculated based on the total number of vesicles (dots) per image divided by the number of cells per image. The term ‘cell’ is used instead of ‘confocal cell section’. Strongly labelled perinuclear regions (marked by dotted circles) were excluded from vesicle counting. Zinc imaging Human WT, knockout and mutant TRPML1 fibroblasts were plated on 25 mm glass coverslips in six-well plates or grown in Poly- D -Lysine-coated 1 μ–Slide 8 wells. After 24–48 h, cells were exposed to 100 μM ZnCl 2 in DMEM (with 10% FBS) for 3 h, washed with PBS and incubated with 1 μM FluoZin-3-AM in PBS for 1 h. Cells were subsequently washed with PBS and incubated for 30–60 min in LysoTracker DeepRed/PBS. Cells were washed again with PBS and immediately analysed using a Zeiss confocal laser-scanning microscope (LSM 510). DMSO or MK6-83 were present throughout the experiment. For data quantification, ImageJ software was used. In each experiment, numbers were calculated based on the total number of vesicles (dots) per image divided by the number of cells per image. The term ‘cell’ is used instead of ’confocal cell section’. The minimum particle size was set to three pixels. MTT test for cell viability The MTT test is based on the reductive conversion of MTT into formazan crystals by living cells, which determines mitochondrial activity. Since for most cell populations the total mitochondrial activity is related to the number of viable cells, this assay is broadly used to measure the in vitro cytotoxic effects of drugs on cell lines or primary patient cells. HEK293 cells were maintained in Earle’s Minimum Essential Medium supplemented with 10% fetal calf serum, 2 mM L -glutamine, 100 U ml −1 penicillin and 100 μg ml −1 streptomycin, trypsinised and seeded in poly- L -lysine-coated 96-well cell culture plates at a density of 10 4 cells per well. The following day, medium was exchanged and the test compounds were added. The cytotoxic compounds plumbagin and staurosporine (both 1 μM; Sigma-Aldrich, Germany) and DMSO were included as positive and negative controls, respectively. After 24 h, compounds were removed and cells were incubated with fresh medium, supplemented with MTT (0.5 mg ml −1 ) for 3 h. Subsequently, supernatants were discarded and DMSO was added to lyse the cells and dissolve formazan crystals. Absorbance at 560 and 670 nm was measured in a multiwell plate reader (Polarstar Omega, BMG Labtech; Germany). For statistical analysis, differences of both extinctions were calculated. Statistical analysis All error bars are depicted as s.e.m. Statistical significance was determined via Student’s t -test or one-way analysis of variance followed by Tukey’s post test. Significance is denoted on figures with asterisks as outlined in the legends. All data presented are representative of three or more independent experiments. How to cite this article: Chen, C.-C. et al . A small molecule restores function to TRPML1 mutant isoforms responsible for mucolipidosis type IV. Nat. Commun. 5:4681 doi: 10.1038/ncomms5681 (2014).